p53 destabilizing protein skews asymmetric division and enhances NOTCH activation to direct self-renewal of TICs Tumor-initiating stem-like cells (TICs) are defective in maintaining asymmetric cell division and responsible for tumor recurrence. Cell-fate-determinant molecule NUMB-interacting protein (TBC1D15) is overexpressed and contributes to p53 degradation in TICs. Here we identify TBC1D15-mediated oncogenic mechanisms and tested the tumorigenic roles of TBC1D15 in vivo. We examined hepatocellular carcinoma (HCC) development in alcohol Western diet-fed hepatitis C virus NS5A Tg mice with hepatocyte-specific TBC1D15 deficiency or expression of non-phosphorylatable NUMB mutations. Liver-specific TBC1D15 deficiency or non-p-NUMB expression reduced TIC numbers and HCC development. TBC1D15–NuMA1 association impaired asymmetric division machinery by hijacking NuMA from LGN binding, thereby favoring TIC self-renewal. TBC1D15–NOTCH1 interaction activated and stabilized NOTCH1 which upregulated transcription of NANOG essential for TIC expansion. TBC1D15 activated three novel oncogenic pathways to promote self-renewal, p53 loss, and Nanog transcription in TICs. Thus, this central regulator could serve as a potential therapeutic target for treatment of HCC. Chronic heavy alcohol consumption is a major health issue worldwide. Excessive alcohol consumption causes alcoholic liver disease, which progresses from fatty liver to alcoholic steatohepatitis, cirrhosis, and ultimately hepatocellular carcinoma (HCC). The International Agency for Research on Cancer designates alcohol as a type 1 carcinogen [1] . Thus, elucidation of the cellular and molecular mechanism(s) by which alcohol initiates and promotes tumor development will undoubtedly help establish useful therapeutic strategies. Tumor-initiating stem-like cells (TICs) are the “root cause” of cancer—the cells that achieve self-renewal, cancer progression, tissue invasion, metastasis, chemoresistance, and recurrence after chemotherapy [2] . Although TICs are identified in different types of cancers and represent a hallmark of therapy-resistance [3] , there is no coherent understanding of the underlying mechanisms for their unchecked proliferation, tumorigenic activity, and clinical intractability. Our studies revealed that specific ectopic expression of TLR4 in hepatocytes [4] of transgenic HCV NS5A mice [5] and activation by endotoxemia associated with alcohol consumption, leads to tumor formation [6] . This occurs via induction of stem cell factor NANOG and generation of NANOG+/CD133+ TICs [6] , [7] , [8] . Such CD133+ TICs have also been isolated from three other HCC animal models and patient HCC tissues and were characterized by their NANOG-dependent self-renewal and tumor-initiating activities [6] , [7] , [8] . Activation of NANOG occurs by leptin receptor OB-R-mediated OCT4 and SOX2 upregulation [9] , TWIST induced by NANOG with STAT cooperation [8] , and NANOG-driven mitochondrial metabolic reprogramming [7] . The oncogenic role of TLR4 activated by endotoxin has been confirmed by others in a different liver tumor model [10] . The stem cell population is maintained by asymmetric divisions in which one daughter cell commits to specific fate and the other maintains parental pluripotency. The p53 interacting partner protein NUMB (homology of numb protein) preserves this intrinsic cellular asymmetry by preventing ubiquitin-mediated proteolysis of p53 catalyzed by the MDM2 E3 ubiquitin ligase [11] . Therefore, NUMB serves as an important barrier against pluripotency and the unlimited expansion of TICs [9] . We recently showed that NANOG-mediated induction of Aurora A kinase (AURKA), an upstream kinase for aPKCζ, and repression of Lethal Giant Larva 2 (LGL2 or LLGL2), an aPKCζ inhibitor, leads to aPKCζ upregulation and activation. This in turn results in aPKCζ-mediated NUMB phosphorylation, NUMB dissociation from p53, and p53 degradation (Fig. 1a ) [12] . We also identified a fresh NUMB-interacting protein, TBC1D15 (Tre2/Bub2/Cdc16 Domain Family Member 15) which is overexpressed and contributes to p53 degradation in TICs [9] . This gene encodes a member of the Ras-like protein in the superfamily of brain-GTPase-activated proteins that share the conserved Tre-2/Bub2/Cdc16 domain. TBC1D15 acts as a mitochondrial Rab GTPase-activating protein (Rab-GAP), and can affect autophagy organism development and morphology downstream of Parkin activation. TBC1D15 is recruited by mammalian Fist1, which is a mitochondrial receptor that functions in the regulation of mitochondrial morphology [13] , [14] . TBC1D15 also has been identified as Rab7 GAP in vivo and in vitro, and can modulate lysosomal morphology [15] , [16] . In addition to interacting with Rab7, TBC1D15 is required for RhoA accumulation during membrane blebbing and cytokinesis [17] . In the present study, we demonstrate that NUMB phosphorylation and TBC1D15 (containing the cell fate determinant Canoe homology domain that is essential to the asymmetric cell division machinery) are mutually required for liver tumorigenesis in vivo. We also show that TBC1D15 interacts with the asymmetric division machinery to disrupt its function, initiate p53 degradation and self-renewal, and cooperates with the Notch pathway to promote tumorigenesis. Fig. 1: TBC1D15 inhibits hepatocyte differentiation, maintain symmetric cell division, and promotes oncogenesis. a Hypothetical model. Novel NUMB-binding protein TBC1D15 promotes NUMB phosphorylation and p53 degradation. b Targeted disruption of mouse Tbc1d15 gene by Cre-LoxP system. c Schematic illustrations of how tumor incidence and tumor growth in Alb::CreERT2;Tbc1d15 FL/FL ;NS5A vs Tbc1d15 FL/FL ;NS5A mice. d The incidence was reduced in TBC1D15 deficient hepatocytes mice. Error bars represent ±SEM. p Values are shown from a chi-square test * p = 0.000465 (chi-square test). e Ratio of tumor mass over liver mass (%) was decreased in TBC1D15 deficient hepatocytes mice. Error bars represent ±SEM. p Values are shown from a chi-square test. * p = 0.000229 (Student’s t test). f (left) Immunostaining showed Vimentin and AFP expression in liver tumor tissues. Scale bar, 30.32 μm. (right) H&E staining displayed HCC histology. g Immunoblots of liver proteins from TBC1D15 deficient hepatocytes mice. h (top) The percentage of CD133+/CD49f +/CD45− TICs in total tumor cells determined by FACS analysis. The percentage of TICs of tumor cells were calculated as mean ± SD ( n = 3). * p = 0.00047 (Student’s t test). (bottom) Spheroid formation of Isolated CD133+/CD49f+/CD45− TICs. Spheroid numbers were counted as mean ± SD ( n = 3). * p < 0.01 (Student’s t test). i Schematic illustrations of how tumor incidence in vector and adenovirus-based Cre expression in ES cells. j Expression of a N-TBC1D15 was validated by immunoblot analysis. k Hepatocyte differentiation makers, Albumin and HNF4A measured by qRT-PCR, show marked downregulations by N-TBC1D15 expression. Data are represented as mean ± SEM ( n = 4). p -Values by two-tailed unpaired t test. * p < 0.0001 (Student’s t test). l Tumor incidence was increased in the mice implanted with ES cells expressing N-TBC1D15. Error bars represent ±SEM. p -Values by two-tailed unpaired t test. * p = 0.007313 (chi-square test). m (top) Schematic illustrations of how asymmetrical vs symmetrical division controlled by NUMB and TBC1D15. (bottom) Immunofluorescence analyses of TICs. Scale bar, 10 μm. n , o The percentage of asymmetrical vs symmetrical division in TBC1D15 knockdown, overexpression of TICs ( n ) and in Nanog knockdown of normal hepatoblasts isolated from fetal mouse livers ( o ). The representative pictures are shown from three independent experiments. Oblique: ambiguous phenotype between asymmetric and symmetric cell division. Source data are provided as a Source Data file. Full size image Liver-specific deletion of TBC1D15 attenuates p53 loss We tested first if hepatocyte-specific TBC1D15 deficiency prevented loss of p53 and liver tumor development by using the inducible Alb::CreERT approach described above (Fig. 1b ). We generated NS5A Tg mice carrying a floxed Tbc1d15 locus (Supplementary Fig. 1 ) which allowed tamoxifen-inducible, hepatocyte-specific ablation of this gene ( Alb::CreERT;Tbc1d15 f/f ;NS5A ) (Fig. 1c ). Liver tumor incidence in wild type Tbc1d15 f/f ;NS5A mice after 12 months of alcohol-Western diet feeding was 50%, which was reduced significantly to 16% in TBC1D15-deficient hepatocytes of Alb::CreERT;Tbc1d15 f/f ;NA5A mice (Fig. 1d ). Incidence of liver tumor (left) and tumor pictures (right) of the four genetic groups of mice (Fig. 1d ). Mouse tumors have vimentin and AFP expression (Fig. 1f ). This genetic manipulation also reduced tumor mass (Fig. 1e ) and abrogated NANOG upregulation, phosphorylation of NUMB, and p53 loss in these livers (Fig. 1g ). In addition, the percentage of CD133+ TICs in total tumor cells of Alb::CreERT2;Tbc1d15 f/f ;NA5A mice was decreased by 70% (Fig. 1h , top). These TICs exhibited reduced self-renewal activity in vitro (Fig. 1h , bottom), as compared to CD133+ TICs from the Tbc1d15 f/f ;NA5A mice. These results underscored the requirement of hepatocyte TBC1D15 for liver tumor development and the generation of TICs in this animal model. N-terminus of TBC1D15 protein inhibits differentiation We previously showed that the N-terminal region of TBC1D15 (N-TBC1D15, aa 2–158) containing the 50 aa Canoe homology domain is indispensable for NUMB association and p53 degradation [9] . We examined if the overexpression of N-TBC1D15 inhibited hepatocyte differentiation and promoted oncogenic transformation of ES cells. This was accomplished using a Cre-activated N-TBC1D15 LSL ( LSL: Lox-Stop-Lox) expression vector (Fig. 1i ) confirmed by immunoblotting (Fig. 1j ). Differentiation-induction medium upregulates hepatocyte-specific genes such as Albumin or Hnf4a in ES cells. However, N-TBC1D15 expression inhibited induction of these hepatocyte genes (Fig. 1k ). ES cells (with or without expression of N-TBC1D15) were cultured in the hepatocyte differentiation medium, then implanted subcutaneously into NOG TM mice, and tumor development was examined for 60 days. Mice with tumors greater than 25 mm 3 were recorded as positive. These N-TBC1D15 overexpressing cells cultured in the differentiation-induction medium prior to transplantation into NSG TM mice formed tumors at an 80% incidence rate. By contrast control cells lacking N-TBC1D15 expression rarely produced tumors (~10%) (Fig. 1l ). These results demonstrated that the overexpression of N-TBC1D15 alone is sufficient to suppress hepatocyte differentiation and confer tumorigenic activity in ES cells. Next, we tested how TBC1D15 regulated NUMB-dependent asymmetric division. CD133+ TICs isolated from the alcohol Western diet-fed Ns5a Tg mice showed symmetric localization of the polarity protein NUMB [18] , [19] . This was demonstrated by reduced polarization of fluorescent NUMB, which is indicative of the loss of asymmetric division. TBC1D15 knockdown (KD) in TICs restored cell polarization of NUMB while TBC1D15 overexpression (OE) supported the symmetry of NUMB localization (Fig. 1m and Supplementary Fig. 2c ). Silencing of TBC1D15 is correlated with a loss of cell division asymmetry as demonstrated by symmetric cell distribution of LGN (Fig. 1m ). TBC1D15 KD in TICs reduced the percentage of TICs showing symmetric division and reciprocally increased asymmetric cell division while TBCD1D15 OE resulted in the opposite effect (Fig. 1n ). Nanog KD reduced the percentage of TICs undergoing symmetrical division approaching that observed in mouse hepatoblasts (Fig. 1o ). These results validated the pivotal role of TBC1D15 in TIC symmetric cell division. TBC1D15 interacts with NuMA1 and prevents NuMA1–LGN interaction While we have shown TBCD1D15 was required for p53 degradation facilitated by NUMB phosphorylation, the mechanism by which TBC1D15 regulates NUMB phosphorylation is unknown. To this end, we searched for in vivo partners of TBC1D15-mediated regulation by large-scale immunoaffinity purification of interacting proteins of endogenous TBC1D15 in TICs and Identification of interaction partners was accomplished by liquid chromatography–tandem mass spectrometry (LC–MS/MS: Fig. 2a and Supplementary Fig. 2a, b ). This approach identified several high-confidence interacting proteins, including NuMA1, NOTCH1/2/3/4, and RANGAP1 (Fig. 2a and Supplementary Figs. 2 and 3 ). These candidates were also present in the enriched pathway analysis developed from the MS data for TBC1d15 immunoaffinity purified products (Supplementary Fig. 4 ). Co-IP-Western blot analysis of cell lysates confirmed that TBC1D15 interacted with NuMA1 and RANGAP1 (Fig. 2b ). RANGAP1 regulates RAN GTPase activity, expression of AURKA and mitosis [20] . NuMA1 binds LGN and Dynein to assemble an asymmetric cell division machinery complex. Indeed, 3D computer modeling predicted TBC1D15 would bind NuMA1 (Fig. 2c and Supplementary Fig. 5 ). Based on the domain section of NuMA, NuMA aa 1788 to the end portion was simulated into the structure. The TBC1D15 of this structure is used to dock with NuMA from 3ro2 with LGN. In silico analysis reveals TBC1D15 binds a domain of NuMA1 that also binds LGN, suggesting a competition between them for binding with NuMA1. TBC1D docked to NUMA with further alignment of LGN (3ro2), showing partial competition for the binding site of NUMA (Fig. 2c , bottom). Fig. 2: TBC1D15–NuMA1 interaction inhibits asymmetric cell division via inhibition of key asymmetric machinery, NuMA1–LGN interaction. a Shotgun LC–MS/MS was performed on immunoaffinity purified TBC1D15-interacting proteins (highlighted in red boxes; NuMA1, RANGAP1, and NOTCH1, 2, 3, 4). b Co-immunoprecipitation-immunoblot analysis confirmed that TBC1D15 interacts with NOTCH1/2, NuMA1, and RANGAP1. c In silico analysis predicts an interaction between TBC1D15 and NuMA1. (top) Structure model of TBC1D15 (green) binding NuMA1 (blue). (middle) Docking between TBC1D15 and NuMA1 was simulated. (bottom) TBC1D docked to NUMA with further alignment of LGN (3ro2), showing partial competition for the binding site of NUMA. TBC1D15 in green, LGN in blue, and partial NUMA in yellow. d Human TBC1D15 protein has 51% homology with Drosophila cell fate determinant Canoe (SNO: Mammalian AFADIN homologue) that binds mammalian homologue of LGN ( Drosophila Pins). e IP-Western blot analysis (left panel) and reverse IP-Western blot analysis (right panel) were performed in TBC1D15 overexpression. f Domain mapping of TBC1D15 binding domain of NuMA1 by using GFP-fused NuMA1 truncation or mutant proteins and Flag-tagged TBC1D15. g The binding of purified flag-TBC1D15 protein with or without purified GFP-NuMA1 mutant protein was tested by in vitro binding assay. h We performed FRET analyses between TBC1D15-CFP and NuMA1-YFP. (left upper panel) Cartoon depicting binding partners TBC1D15 and NuMA1 tagged with fluorescent proteins CFP and YFP. (left bottom panel) Living CD133+ cells transfected with the controls CFP only, YFP only, CFP and YFP as well as the CFP–YFP fusion proteins were analyzed on a FACS flow cytometer. (right panel) Representative optical images showed CFP and YFP expression in CD133+ cells with CFP and YFP. CFP is shown in red and YFP in green (Supplementary Fig. 10 ). i Hypothetical model of TBC1D15-mediated disruption of the interaction between NuMA and LGN that inhibits asymmetric cell division and promotes symmetric cell division. Source data are provided as a Source Data file. Full size image From in silico structural simulations of NuMA1, T1804 was more important than S1969 of NuMA1 C-terminal fragment for mediating an interaction with the N-terminal domain (aa 1–270) of TBC1D15. The G168 residue of TBC1D15 (green) interacted with T1804 of NUMA (blue) (Fig. 2c , bottom). Human TBC1D15 protein has 51% homology to Drosophila cell fate determinant Canoe (CNO) (Fig. 2d ) that binds mammalian homologue of Pin (LGN) [21] . Furthermore, NuMA1 interaction with LGN was suppressed by TBC1D15 as shown by co-IP-Western blot analysis (Fig. 2e , left panel) and reverse co-IP-Western blot analysis (Fig. 2e , right panel). These results demonstrate that TBC1D15–NuMA1 interaction potentially prevents interaction between NuMA1 and LGN. These results indicated that TBC1D15 interacts with NuMA1 to prevent NuMA1–LGN interaction (Fig. 2e ). To map a TBC1D15 interaction site of NuMA1, we generated GFP-fused NuMA1 proteins with truncations and mutations to test their interactions with Flag-tagged TBC1D15 (Fig. 2f ). The GFP-NuMA1 C-terminus (aa 1700–2115), but not the N-terminus (aa 1–213) interacted with TBC1D15. This C-terminal region contains S/T residues including serine or threonine residue which are phosphorylated by AURKA resulting in dissociation from LGN and a loss of cell division symmetry [22] . Alanine substitutions of three such residues (GFP-NuMA1 C-3A) largely abrogated the NuMA1 interaction with TBC1D15, suggesting the importance of serine or threonine phosphorylation for TBC1D15’s interaction with the NuMA1 C-terminus for disrupting asymmetric cell division control. We performed new experiments and have added the in vitro binding assay of TBC1D15 and NuMA1 (wild-type or T1804A, S2047A, and T1991A mutation). Actually, in this manuscript, we tested a single alanine substitution of T1804 (NuMA1 T1804A). And we suggested that the importance of T1804 phosphorylation for TBC1D15’s interaction with the NuMA1 C-terminus for disrupting asymmetric cell division control in Fig. 2i . We examined alanine substitutions of S2047A, T1991A, and T1804 (Fig. 2g ). To measure FRET signals by FACS, CD133 positive cells expressing either the cyan fluorescent protein (CFP) and/or yellow fluorescent protein (YFP) were analyzed (Fig. 2h , top). Compared to cells transfected with 40% positive control cells transfected with a CFP–YFP fusion protein, only 10% of cells co-transfected with CFP and YFP were recorded as FRET positive (Fig. 2h , right). We speculated that the TBC1D15–NuMA1 interaction potentially prevents interaction between NuMA1 and LGN, thus leading to inhibition of asymmetric cell division (Fig. 2j , left). This model TBC1D15 structure was used to dock to the NuMA1–LGN complex (Fig. 2j , right). Indeed, this 3D conformational modeling predicted that TBC1D15 would partially occupy the LGN position with NuMA1 (PDB 3ro2 ) (Supplementary Fig. 5 , right). Translational relevance of TBC1D15 We sought to determine the translational relevance of the tumor promotion activity of TBC1D15 as described in the present studies. For this, the TCGA liver cancer data were analyzed for expression of TBC1D15 and NOTCH1 in relation to HCC stage. These data showed co-overexpression of these two proteins was highest in the late metastatic stage as compared to normal or earlier stages of HCC, suggesting a role for the tumor-promoting TBCD1D15–NOTCH interaction (Fig. 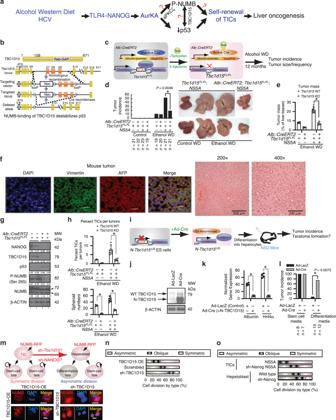Fig. 1: TBC1D15 inhibits hepatocyte differentiation, maintain symmetric cell division, and promotes oncogenesis. aHypothetical model. Novel NUMB-binding protein TBC1D15 promotes NUMB phosphorylation and p53 degradation.bTargeted disruption of mouseTbc1d15gene byCre-LoxPsystem.cSchematic illustrations of how tumor incidence and tumor growth inAlb::CreERT2;Tbc1d15FL/FL;NS5AvsTbc1d15FL/FL;NS5Amice.dThe incidence was reduced in TBC1D15 deficient hepatocytes mice. Error bars represent ±SEM.pValues are shown from a chi-square test *p= 0.000465 (chi-square test).eRatio of tumor mass over liver mass (%) was decreased in TBC1D15 deficient hepatocytes mice. Error bars represent ±SEM.pValues are shown from a chi-square test. *p= 0.000229 (Student’sttest).f(left) Immunostaining showed Vimentin and AFP expression in liver tumor tissues. Scale bar, 30.32 μm. (right) H&E staining displayed HCC histology.gImmunoblots of liver proteins from TBC1D15 deficient hepatocytes mice.h(top) The percentage of CD133+/CD49f +/CD45− TICs in total tumor cells determined by FACS analysis. The percentage of TICs of tumor cells were calculated as mean ± SD (n= 3). *p= 0.00047 (Student’sttest). (bottom) Spheroid formation of Isolated CD133+/CD49f+/CD45− TICs. Spheroid numbers were counted as mean ± SD (n= 3). *p< 0.01 (Student’sttest).iSchematic illustrations of how tumor incidence in vector and adenovirus-based Cre expression in ES cells.jExpression of a N-TBC1D15 was validated by immunoblot analysis.kHepatocyte differentiation makers,AlbuminandHNF4Ameasured by qRT-PCR, show marked downregulations by N-TBC1D15 expression. Data are represented as mean ± SEM (n= 4).p-Values by two-tailed unpairedttest. *p< 0.0001 (Student’sttest).lTumor incidence was increased in the mice implanted with ES cells expressing N-TBC1D15. Error bars represent ±SEM.p-Values by two-tailed unpairedttest. *p= 0.007313 (chi-square test).m(top) Schematic illustrations of how asymmetrical vs symmetrical division controlled by NUMB and TBC1D15. (bottom) Immunofluorescence analyses of TICs. Scale bar, 10 μm.n,oThe percentage of asymmetrical vs symmetrical division in TBC1D15 knockdown, overexpression of TICs (n) and in Nanog knockdown of normal hepatoblasts isolated from fetal mouse livers (o). The representative pictures are shown from three independent experiments. Oblique: ambiguous phenotype between asymmetric and symmetric cell division. Source data are provided as aSource Datafile. 3a and Supplementary Table 1 for Box plot statistics). Based on this meta-analysis we examined the expression of NANOG, TBC1D15, p53, N1ICD, and p-(S265) NUMB in liver protein extracts of normal human subjects vs patients with alcoholic cirrhosis/hepatitis (Fig. 3b, c ). Hypothetical model of TBC1D15-mediated NOTCH activation and stabilization leading to NICD-dependent transactivation of the Nanog gene to generate TICs, leading to HCC development. Normal liver progenitor cells (LPC) differentiate into either cholangiocytes or hepatocytes through NOTCH signaling or NUMB-mediated signaling, respectively (Fig. 3c ). This expression signature was associated with a high propensity for liver cancer development (Fig. 3b ). The results clearly demonstrated the coordinated upregulation of NANOG, TBC1D15, N1ICD, and p-(S265) NUMB with p53 depletion in these patients. From this analysis, we concluded that TBC1D15 was an important mediator in two oncogenic pathways (loss of p53 and NOTCH activation). Fig. 3: TBC1D15–NOTCH1 interaction promotes self-renewal and oncogenesis. a Late stage HCC patients exhibit higher NOTCH1 and TBC1D15 combined expression (TCGA): Each circle represents the expression of a single sample ( p < 0.0001). b Explant liver tissues from alcoholic cirrhosis/hepatitis patients (immunoblots). c Hypothetical model. d Co-IP-Western blot analyses confirmed the interaction of TBC1D15 with full-length NOTCH1/2/3/4. e Immunoblot analyses performed expression of NOCH1 and N1ICD in TICs and primary hepatocytes. f CD133+ Huh7 cells express a higher level of N1ICD compared to CD133− cells (immunoblot). g TBC1D15 overexpression elevated N1ICD in PH5CH cells (immunoblot). h Colony formation (left) and expression of Nanog mRNA (right) in TBC1D15, sh-Scramble, and sh-NOTCH expressing PIL4 cells. Colony numbers were calculated as mean ± SD ( n = 3). [left; * p = 0.00145 (TBC1D15 vs sh-NOTCH); ** p = 0.0056 (Vector vs TBC1D15); ** p = 0.01668 (sh-Scramble vs sh-NOTCH); Student’s t test]. p -Values by two-tailed paired t test. [right; * p = 0.004988 (TBC1D15 vs sh-NOTCH); ** p = 0.002575 (Vector vs TBC1D15); ** p = 0.02014 (sh-Scramble vs sh-NOTCH); Student’s t test]. i TBC1D15 KD abrogated the activity of HEY1 promoter-luciferase in Huh7 cells. Data are represented as ±SD ( n = 4). p -Values by two-tailed paired t test. * p = 0.00953 (shTBC1D15 vs sh-Scramble; Hey1); * p = 0.018604 (sh-TBC1D15 vs sh-Scramble; Δ215); Student’s t test. j CSL-mediated Nanog activation. k Six mutant-luciferase constructs. Data are represented as ±SD ( n = 3). p -Values by two-tailed paired t test. * p = 0.008879 (WT vs M1); * p = 0.000117 (WT vs M2); * p = 0.000262 (WT vs M3) (Student’s t test). l TBC1D15 or NOTCH1 expression promotes hepatoblast proliferation. Data are represented as ±SD ( n = 4). p -Values by two-tailed paired t test. * p = 0.0001149 (Vector vs TBC1D15); ** p = 0.00001853 (Vector vs NOTCH1; Student’s t test). mTBC1D15 KD reduced N1ICD but increased NOTCH1 in Huh7 cells. m CD133+ Huh7 cell lysates were analyzed for immunoblots in the presence of shRNA targeting TBC1D15 or scrambled shRNA. TBC1D15 KD reduced N1ICD but increased NOTCH1 in Huh7 cells. n Tumor growth after TIC transplantation in NSG TM mice is suppressed by TBC1D15 KD. Error bars represent ±SEM. o Tumor volume determined 2 months after transplantation of TICs into NSG TM mice. Error bars represent ±SEM ( n = 4). p -Values by two-tailed unpaired t test. * p = 0.00000233 (NICD vs shTBC1D15); ** p = 0.0000181 (sh-Scramble vs NIICD) (Student’s t test). p TBC1D15 KD reduced NOTCH1 stability. NOTCH1 protein was immunoprecipitated and detected by immunoblotting (left). The NOTCH1 autoradiographic reading (right). Source data are provided as a Source Data file. Full size image TBC1D15 interacts with NOTCH to activate NOTCH pathway Our immunoaffinity purification for TBC1D15 interacting proteins, identified NOTCH1, 2, 3, and 4 as high-confidence interacting proteins (Supplementary Fig. 4 ). Co-IP-Western blot analysis of TIC cell lysates confirmed TBC1D15 interacted with all NOTCH isoforms in both full length and activated NICD forms (Fig. 3d ). TICs expressed cleaved NICD while primary hepatocytes expressed full-length NOTCH1 (Fig. 3e ). Sorted CD133+ Huh7 cells also expressed activated NOTCH 1 (NICD) while CD133− cells only expressed the full-length NOTCH1 (Fig. 3f ). This suggested NOTCH pathway activation occurred in tumorigenic CD133+ cells. To test the effects of TBC1D15 OE on full length NOTCH1 and N1ICD levels, we used non-transformed cell line PH5CH, which has no or minimal N1ICD (Fig. 3g , lane 2). TBC1D15 OE resulted in increased N1ICD (Fig. 3g , lane 1). To dissociate the effect of NOTCH1 activation, we treated the cells with the γ-secretase inhibitor DAPT and repeated the same TBC1D15 OE in PH5CH cells. Under this condition, both full-length NOTCH1 and N1ICD were evidently increased (Fig. 3g , lane 3), consistent with TBC1D15 stabilization of NOTCH1/N1ICD and/or activation of NOTCH1 in a manner independent of γ-secretase [23] . DAPT, an inhibitor of the γ-secretase complex, indirectly inhibits the pathway of Notch, a key target of γ-secretase. A γ-secretase inhibitor prevents proteolytic cleavage of the Notch intracellular domain (NICD), which is necessary for the Notch signaling response when NICD translocate to the nucleus and affect transcription [24] , [25] . Although we demonstrated TBCD1D15-facilitated p53 degradation and TIC self-renewal in other liver cell lines, we noticed that the loss of p53 occurred only in hepatoblasts (PIL4 cells) and failed to result in transformation. Transformation independent of p53 was observed when TBC1D15 was expressed in these cells leading to increased self-renewal (colony formation) (Fig. 3h , left) and higher NANOG expression (Fig. 3h , right). We tested if these effects required the NOTCH pathway. Indeed, NOTCH1 KD significantly attenuated the observed transformation effects of TBCD1D15 in these cells (Fig. 3h ). To examine the functional relationship of the NOTCH pathway to TBC1D15, we knocked down TBC1D15 (TBC1D15 KD) in Huh7 cells. This manipulation caused a loss of HEY1 -promoter activity, the conventional readout of NICD transactivity (Fig. 3i ), indicating that TBC1D15 enhances activation of a NOTCH target gene. Novel CSL sites in Nanog gene We have previously shown that TIC self-renewal and tumorigenic activity require NANOG which is transcriptionally induced by TLR4 signaling in part via E2F1 [7] , However, even without LPS-TLR4 stimulation, TICs maintain the self-renewal phenotype, indicating that TICs possess an intrinsic mechanism to promote transcription of this stemness gene. Using the bioinformatics tools, we have identified a previously unreported CSL/RBPJ site for binding NICD in the proximity of the OCT4/SOX2 binding element of Nanog promoter (−212/−119) (Fig. 3j ). Additionally, a functionally important E2F1 binding site is found within the distal enhancer, 5 kb upstream of the transcription initiation site (TSS) of Nanog gene [7] , [26] . Just downstream of this E2F site, we have identified a second CSL/RBPJ sequence element (see Fig. 3j ). We characterized the functionality of these two putative CSL sites in Nanog for transcriptional activity. Two regions together may account for majority of the reporter activity, including the enhancer region (−5421/−4828) containing the E2F1 and CSL elements and the TSS proximal promoter region (−153/+1) containing the CSL and OCT4/SOX2 sites [7] . Mutations in CSL elements reduced Nanog promoter luciferase activities, indicating that CSL binding sites in these regions are critical for Nanog promoter activities. The overexpression of TBC1D15 or NOTCH1 increases hepatoblast proliferation (Fig. 3l ). Freshly-isolated TICs transduced with shRNA lentivector were transplanted subcutaneously into NSG mice forming a growing tumor which was reduced in size by more than 80% upon TBC1D15 KD (Fig. 3m, n ). Concomitant expression of Notch 1 intracellular domain (N1ICD), partially rescued this inhibition of tumor growth (Fig. 3n ). Conversely, N1ICD expression alone resulted in a significant increase in tumor growth promotion that was attenuated by TBC1D15 KO (Fig. 3n ) to the level below the growth achieved in control TICs (Fig. 3n, o ). These results indicated TBC1D15 has NICD-dependent and -independent tumor promoter activities, and that the NICD-dependent effect is at a level downstream of NOTCH activation. We examined the cooperative relationship between TBC1D15–NOTCH/N1ICD in a more physiologic context. PIL4 hepatoblasts with or without lentivirus-based N1ICD expression and/or Tbc1d15 KD were orthotopically transplanted into the left liver lobe of NSG mice. PIL4 cells expressing N1ICD expression formed large tumors within 2 months of transplantation, but TBC1D15 KD in these cells significantly reduced this growth, confirming that the N1ICD tumor promotion effect required TBC1D15 (Fig. 3n, o ). These results were consistent with the model that TBC1D15 rendered tumorigenic effects partly via its ability to activate NOTCH and to support N1ICD activity. In support of this mode of NOTCH activation, TBC1D15 knockdown in Huh7 cells diminished N1ICD levels in favor of increased levels of full-length NOTCH-1 (Fig. 3m ). A mechanism by which TBC1D15 supports NICD activity is by stabilization of N1ICD. To test this possibility, we examined N1ICD protein stability in Huh7 cells stably transfected with shRNA for TBC1D15 vs scrambled shRNA. Cells were radiolabeled with 35 S-methionine and whole cell lysates were prepared at timed intervals following cycloheximide treatment. This analysis showed that labeled N1ICD protein was detected in cells when transduced with scrambled shRNA with a half-life of 162 min (Fig. 3p ). By contrast, the cells treated with sh-TBC1D15, mainly showed labeled full-length NOTCH-1 but very little N1ICD that was more rapidly degraded with a half-life of 88 min. These results indicated that TBC1D15 promoted NOTCH-1/N1ICD stability by specific TBC1D15–NOTCH interaction. NOTCH1–TBC1D15 interaction domains We next performed domain mapping studies to define a TBC1D15 interaction site of NOTCH1 by using deletion mutants (Fig. 4a ). We tested the ability of wild-type NOTCH1 or a constitutively stable NOTCH1 mutant (PEST domain of NOTCH 1 C-terminal). These mutants lack the constituting the consensus for the E3 ubiquitin-ligase FBW7A, the major negative regulator of the intracellular NOTCH signal [27] , [28] . This analysis demonstrated that TBC1D15 interacted with NOTCH1/N1ICD within a region spanning aa 2171–2473 of the C-terminal PEST domain known for the initiation of protein degradation [29] (Fig. 4a, b ). Note Myc-tagged TBC1D15 interacted with intact N1ICD-HA and N1ICD with a partial deletion of the PEST domain distal to aa 2473: N1ICDΔPEST (aa 1754–2473) but not with N1ICD with a complete deletion of the PEST domain: N1ICDΔPEST (aa 1754–2171) (Fig. 4b ). In fact, NUMB is known to bind this PEST domain to recruit the E3 ubiquitin ligases, ITCH and FBW7 for ubiquitination and subsequent degradation of NOTCH1 and N1ICD (Supplementary Fig. 8 ) [30] . As TBC1D15 interacts with NUMB, our results suggested that TBC1D15 interfered with NUMB-mediated NOTCH/N1ICD degradation by binding to the same PEST domain. Fig. 4: NOTCH1 C-terminal PEST domain interacts with N-terminus of TBC1D15 for cooperative oncogenic activity. a Scheme representation of NOTCH-1 deletion mutants were generated. Co-IP-Western blot analysis identified a region between aa 2171 and aa 2473 of the PEST domain as the interaction site. b Co-IP-Western blot analysis identified interaction domains of TBC1D15 interacted with intact N1ICD-HA and N1ICDΔPEST (aa 1754–2473). c The N-terminus but not C-terminus of TBC1D15 interacts with NOTCH-1. A similar domain mapping of TBC1D15 for its interaction with NOTCH-1 revealed aa 1–200 N-terminal fragment with known lysine residues for ubiquitination (Myc-HA-TBC1D15-N term) but not the C-terminus (Myc-HA-TBC1D15-C term), interacted with NOTCH-1. Substitution of these lysines with arginine (Myc-HA-TBC1D15-N 2KR) did not affect the binding. d Co-IP/IB showed TBC1D15–NOTCH1 interaction was lost by deletion of the N-terminus interacting domain (ΔN) while the TBC1D15–NUMB interaction was lost by deletion of the CNO domain (ΔCNO). NICD expression was lost when TBC1D15 with ΔN was expressed while p53 was restored when TBC1D15 with ΔCNO was expressed. This underscored the importance of these distinct domains for the two respective functions. e Additional deletion analysis revealed the N-terminal domain spanning aa.163–217 upstream of the NUMB-binding Canoe (CNO) domain (aa.218–270) was responsible for TBC1D15 interaction with NOTCH. f ΔCNO, ΔN, or both domains of TBC1D15 was reduced spheroid formation of PH5CH cells. Spheroid numbers were counted as mean ± SD ( n = 4). p -Values by two-tailed unpaired t test. ** p = 0.0001544 (Vector vs TBC1D15); * p = 0.0002660 (TBC1D15 vs ΔCNO); * p = 0.00008665 (TBC1D15 vs ΔN); * p = 0.00035214 (ΔCNO vs ΔN) (Student’s t test). g ΔCNO, ΔN, or both domains incrementally contributed to the abrogation of TBC1D15-induced tumor formation (tumor pictures; left/middle and tumor volumes; right) in NSG TM mice. The visible tumors were measured at the indicated days, Error bars represent ±SD ( n = 4). p -Values by two-tailed unpaired t test. ** p = 0.00001448 (Vector vs TBC1D15); * p = 0.00003475 (TBC1D15 vs ΔCNO); * p = 0.00001831 (TBC1D15 vs ΔN); * p = 0.00009508 (ΔCNO vs ΔN) (Student’s t test). Source data are provided as a Source Data file. Full size image We performed the reciprocal structure mapping of TBC1D15 to identify its interacting domain with NOTCH/NICD. The N-terminal (aa 1–200) but not a C-terminal fragment of TBC1D15 was found to bind NOTCH1 (Fig. 4c ). The TBC1D15 N-terminal fragment has two lysine residues identified as ubiquitination sites for the initiation of degradation [9] . A degradation-resistant mutant with these two lysine residues replaced with arginine (myc-HA-TBC1D15-N-2KR), also interacted with NOTCH-1 (Fig. 4c ). Further deletion analysis of TBC1D15 within the N-terminus revealed a domain spanning aa 218–270 distinct from the NUMB-binding Canoe (CNO) domain (aa 163–217) which interacted with NOTCH/NICD (schematically shown in Fig. 4e ). The latter result also showed that N1ICD interaction was lost when TBC1D15 lacking the NOTCH interacting domain (TBC1D15ΔN or TBC1D15ΔCNOΔN) was expressed and assayed in cell culture, whereas the p53 level was restored when TBC1D15 lacking the CNO domain was expressed (either TBC1D15ΔCNO or TBC1D15ΔCNOΔN) was expressed. Binding of NUMB to this TBC1D15 region was corroborated by co-IP results shown in Fig. 4d . These results confirmed both CNO and NOTCH1 binding domains of TBC1D15 are important for N1ICD expression and p53 turnover. Functional significance of the NOTCH interacting and CNO domains of TBC1D15 was shown by incrementally deletions of TBC1D15 and corresponding reduced spheroid formation (Fig. 4f ) or tumor growth of non-neoplastic immortalized human cell line, PH5CH [31] in NSG mice (Fig. 4g ). By deletion of both NUMB-interacting CNO domain and NOTCH-interacting N-terminal domain in TBC1D15ΔCNOΔN (with possible dominant negative phenotype) we observed maximum suppression of tumor formation, highlighting the importance of these two domains in vivo (Fig. 4g ). RANGAP1–TBC1D15 association promoted NUMB phosphorylation NUMB is phosphorylated at S284 and S265 contributing to the loss of cell division asymmetry [20] . TBC1D15 KD or OE respectively suppressed or increased S265 phosphorylation in Huh7 cells (Fig. 5a ), and these effects correlated with TBC1D15’s ability to regulate aPKCζ activity (Fig. 5c ). However, TBC1D15 KD did not affect protein levels of various kinases that may potentially phosphorylate NUMB, including aPKCζ (Fig. 5b, c ). The ability of TBC1D15’ ability to interact with RANGAP1 suggested that RANGAP1 may positively regulate AURKA and microtubule–kinetochore interaction as previously suggested [13] , which in turn activates aPKCζ for NUMB phosphorylation. This notion was tested by cell-free kinase assay using Huh7 cell lysate and NUMB as a substrate (Fig. 5d ). NUMB phosphorylation was increased by recombinant aPKCζ (raPKCζ) in a dose-dependent manner. NUMB was dose-dependently phosphorylated by recombinant aPKCζ at concentrations up to 1 μM (Fig. 5d(i) ). TBC1D15 enhanced NUMB phosphorylation mediated by aPKCζ and AURKA, and this effect was lost when AURKA is absent. Vector-mediated expression of aPKCζ with or without AURKA expression, only marginally increased NUMB phosphorylation, while concomitant expression of TBC1D15 with AURKA and aPKCζ, conspicuously increased the NUMB phosphorylation. This effect was lost without AURKA expression (Fig. 5d(ii) ), supporting the critical role of TBC1D15–AURKA cooperation in aPKCζ-mediated NUMB phosphorylation. The AURKA inhibitor MK5108 abrogated the TBC1D15–AURKA–aPKCζ cooperative NUMB phosphorylation. In fact, the AURKA inhibitor MK5108 completely abrogated the phosphorylation by this cooperative action of TBC1D15–AURKA–aPKCζ (Fig. 5d(iii) ). This line of regulation was investigated further. We then tested the effect of RANGAP1 expression on the phosphorylation achieved by TBC1D15, AURKA, and aPKCζ. RANGAP1 OE indeed rendered incremental and dose-dependent upregulation of the phosphorylation achieved by TBC1D15–AURKA–aPKCζ (Fig. 5d(iv) ). Conversely, lentiviral RANGAP1 KD by RANGAP1 shRNAs in Huh7 cells prior to in vitro kinase assay, significantly reduced NUMB phosphorylation (Fig. 5d(v) ). Fig. 5: TBC1D15 promotes NUMB phosphorylation through RANGAP1-mediated promotion of AURKA–aPKCζ activation. a TBC1D15 knockdown inhibits NUMB phosphorylation at S265 as demonstrated by immunoblot analysis. b TBC1D15 knockdown or overexpression does not affect kinase protein levels as demonstrated by immunoblot analysis. c TBC1D15 knockdown reduces and TBC1D15 overexpression increases aPKCζ kinase activity demonstrated aby in vitro kinase assays. Data are represented as ±SD ( n = 4). p -Values by two-tailed unpaired t test. * p = 0.00027596 (shTBC1D15 vs shScramble), * p = 0.000008157 (shScramble vs TBC1D15 OE) (Student’s t test). d In vitro cell-free NUMB phosphorylation assay. Each bar represents the mean ± SD of four independent experiments. p -Values by two-tailed unpaired t test. * p = 0.000139 (TBC1D15–AURKA–aPKCζ-NUMB vs AURKA–aPKCζ-NUMB), * p = 0.0002468 (TBC1D15–AURKA–aPKCζ-NUMB vs TBC1D15-aPKCζ-NUMB), * p = 0.00000058 (TBC1D15–AURKA–aPKCζ-NUMB vs TBC1D15–AURKA–aPKCζ-NUMB-0.25μg RANGAP1), * p = 0.00008243 (TBC1D15–AURKA–aPKCζ-NUMB vs TBC1D15–AURKA–aPKCζ-NUMB-0.5 μg RANGAP1), * p = 0.0007145 (TBC1D15–AURKA–aPKCζ-NUMB-shScramble vs TBC1D15–AURKA–aPKCζ-NUMB-shRANGAP1) (Student’s t test). e (top) RANGAP1 knockdown abrogated and RANGAP1 overexpression (OE) enhances AURKA interaction with aPKCζ and TBC1D15 in Huh7 cells as determined by co-IP-Western blot analysis. (bottom) Immunoblot of total cell lysate reveals p-NUMB was reduced by RANGAP1 KD and increased by RANGAP1 OE. PAR6. f We tested if serine or threonine residue of NuMA1 is phosphorylated by Aurora-A, and that this phosphorylation is important for association with TBC1D15. Serine or threonine residue of NuMA1 is phosphorylated by Aurora-A. g Phosphorylation of serine or threonine residue of NuMA1 by Aurora-A is important for asymmetric cell division, judged by immunofluorescence staining of α-Tubulin and NuMA1-GFP intensity. Bar graph represents fold enrichment of GFP-NuMA1. Scale bar, 10 μm. Data are represented as ±SD ( n = 3). p -Values by two-tailed paired t test. * p = 0.000667 (WT vs T1991A) * p = 0.000936 (WT vs S2047A) (Student’s t test). h Hypothetical model that TBC1D15 expression promotes NUMB phosphorylation via RANGAP1–TBC1D15 interaction enhancing AURKA–aPKCζ interaction and activation. Source data are provided as a Source Data file. Full size image To gain mechanistic insights into the observed effects of RANGAP1, we tested if RANGAP1 KD or OE influenced AURKA–aPKC association. Co-IP-Western blot demonstrated that RANGAP1 KD significantly reduced AURKA–aPKC and AURKA–TBC1D15 associations while RANGAP1 OE promoted both associations (Fig. 5e , top). Parallel immunoblotting also showed RANGAP1 KD reduced p-NUMB (Ser265) while RANGAP1 OE significantly increased it (Fig. 5e , bottom), indicating that RANGAP1–TBC1D15 association promoted NUMB phosphorylation by increased interactions among TBC1D15, AURKA, and aPKCζ (Fig. 5f ). We tested if serine or threonine residue of NuMA1 is phosphorylated by Aurora-A, and that this phosphorylation is important for association with TBC1D15. Serine or threonine residue of NuMA1 is phosphorylated by Aurora-A. Phosphorylation of serine or threonine residue of NuMA1 by Aurora-A is important for asymmetric cell division, judged by immunofluorescence staining of α-Tubulin and NuMA1-GFP intensity (Fig. 5f ). The spindle pole in NuMA1 WT vs mutant displayed different degree of NuMA1-GFP intensity. Bar graph represents fold enrichment of GFP-NuMA1. GFP fluorescence intensity was compared in NuMA1 WT vs mutants (Fig. 5g ). These results indicate that TBC1D15–RANGAP1 interaction activated NUMB phosphorylation via TBC1D15–AURKA–aPKCζ-association (Fig. 5h ). Non-phosphorylatable NUMB mutant prevents oncogenesis We next tested the contributory role of NUMB phosphorylation in the genesis of TICs and liver tumors in an HCV Ns5aTg mouse model [5] fed with an alcohol Western diet. Our previous study with NUMB site-directed mutants demonstrates that the triple substitution-mutant of NUMB-3A (carrying non-phosphorylatable S ⇒ A substitutions at S7, S265, S284; see Fig. 6a ) stably binds p53, while the NUMB-3D (S ⇒ D phosphomimetic substitutions at these residues) does not [12] . We used the CRISPR-Cas9 system (Supplementary Figs. 6 , 7 ) to generate transgenic mice to conditionally express in transgenic mice this non-phosphorylatable-mutant NUMB-3A (NUMB-3A) with HA-epitope tag (Supplementary Fig. 6d ). These mice were used for further tumorigenesis studies. This approach enabled a tightly controlled analysis of NUMB-3A mediated effects on the genesis of TICs and liver tumors in Alb::CreERT2;Numb3A LSL ;Ns5a vs Numb-3A LSL ;Ns5a mice (Fig. 6b ). Under normal chow feeding, none of the transgenic mice developed liver tumors, including Ns5a Tg mice. The alcohol-Western diet resulted in a liver tumor incidence of 10% in all transgenic mice strains. NUMB3A expression was notable in that liver incidence was reduced to 5%. By contrast normal chow feeding of these animals did not result in tumor formation (Fig. 6c , left). By comparison, in Numb-3A LSL ;Ns5a mice (without NUMB-3A expression) fed alcohol-Western diet, a 54% incidence of liver tumors was observed after 12 months of feeding. Histological analyses showed that these mice developed HCC (Fig. 6c , bottom) that were positive for Vimentin and AFP (Fig. 6c , bottom right). Fig. 6: Targeted expression of a non-phosphorylatable mutant of NUMB reduces HCC development induced by alcohol-HCV synergism mouse model. a Non-phosphorylatable mutant of NUMB (named as NUMB-3A) was generated by serine-to-alanine substitutions of three NUMB phosphorylation sites. b The experimental strategy of tamoxifen-inducible Cre-mediated NUMB-3A expression using Alb::CreERT2 ; NUMB3A LSL ;NS5A mice. c Incidence of liver tumor (upper left panel), ratio of tumor mass/liver weight (%) (upper middle panel) and liver tumor pictures (upper panel, right) of the four groups of mice was decreased in Alb :: CreERT 2; NUMB3A LSL ; NS5A mice with Ethanol WD. The visible tumors were measured at the indicated days. Error bars represent ±SEM ( n = 3). p Values are shown from a chi-square test * p = 0.0003773 (chi-square test). H&E staining for mouse tumors (bottom left panel). Immunofluorescence staining of Vimentin and AFP in tumor tissues (bottom right panel). Scale bar, 30.32 μm. The representative pictures are shown from three independent experiments. d (top) The percentage of CD133+ TICs in tumor cells is compared among the four different genotypes of mice. (bottom) Tumor volume kinetics of TIC-derived tumors. The percentage of TICs of tumor cells were calculated as mean ± SD ( n = 3). p -Values by two-tailed paired t test. * p = 0.022474 (Student’s t test). e (left) Immunoblots of tumor cell lysates isolated from hepatocyte-specific expression of NUMB-3A mice. (right) Schematic presentations of LPS-activated TLR4 inducing NANOG mediated NUMB phosphorylation for p53 loss and TIC self-renewal, and of NUMB-3A-antagonism of this pathway. f Micro-CT imaging and texture-based VRT were reduced tumor size and tumor volume. The bar graph shows changes in tumor volume before and after the aPKCζ inhibitor. Error bars represent ±SEM. p -Values by two-tailed paired t test. * p = 0.00654 (aPKCζ inhibitor; before vs after treatment), * p = 0.00095 (after treatment; vehicle vs aPKCζ inhibitor) (Student’s t test). g Τhe aPKCζ inhibitor treatment reduced liver tumors spontaneously developed in HCV NS5A Tg mice fed alcohol Western diet as shown by ultrasound sonography. h Immunoblots of tumor cell lysates isolated from NS5A Tg mice fed alcohol WD of the aPKCζ inhibitor vs vehicle. i Summary of oncogenic pathways. NUMB phosphorylation and TBC1D15 are mutually required for liver tumorigenesis. Source data are provided as a Source Data file. Full size image The role of NUMB3 was illustrated by Alb::CreERT2;Numb3A LSL ;Ns5a mice fed the same diet but expressing the mutant NUMB3A. These mice exhibited a significantly reduced tumor incidence of 15%. NUMB-3A overexpression also reduced the average tumor mass by 65% in these mice compared to Numb-3A LSL ;Ns5a mice (Fig. 6c , right). Concomitantly, the percentage of FACS-sorted CD133+CD49f+ TICs decreased by 88% in tumors of Alb::CreERT2;Numb3A LSL ;Ns5a mice (Fig. 6d , top) compared to Numb-3A LSL ;Ns5a mice. Furthermore, the TICs isolated from the former mice exhibited decreased tumor-initiating activity compared to the cells from the latter after transplantation into immunocompromised, recipient NSG mice (Fig. 6d , bottom). Hepatocyte-specific expression of the mutant NUMB-3A in these mice was confirmed by immunodetection which was accompanied by the prevention of p53 loss and NANOG upregulation with attenuated TBC1D15 induction (Fig. 6e , left). These results indicated that tissue-specific (hepatocyte) NUMB phosphorylation indeed contributed to p53 loss and liver tumor development but also resulted in NANOG and TBC1D15 upregulation, suggesting a feed-forward mode of regulation (Fig. 6e , right). Decoy peptide of NUMB phosphorylation reduces tumor size As a complementary approach, tumor-bearing Ns5a Tg mice were fed alcohol-Western diet for 10 months, treated with an aPKCζ inhibitor for 4 weeks and examined for effect by live animal imaging. The inhibitor used to antagonize NUMB phosphorylation is a membrane-permeant, synthetic pseudo-substrate, synthetic peptide, myristoyl-SIYRRGARRWRKL [32] , [33] . As a control, the inhibitor-free vehicle was administered. The aPKC-ζ pseudosubstrate peptide was injected i.p. into the tumor-bearing NS5A Tg mice (50 μmol/mouse, daily, 5 times per week for 4 weeks). Contrast-enhanced microCT and texture-based volume renderings (VRT) were performed to demonstrate a reduction of tumor size and to measure tumor volume based on 3D data collected (Fig. 6f ). This treatment significantly reduced tumor size and volume compared to the vehicle treatment, as assessed by ultrasound sonography and micro-CT imaging (Fig. 6f, g ); thus, this demonstrated the in vivo efficacy of the aPKCζ inhibitor in the context of NUMB activity. Furthermore, immunoblotting of tumor tissues showed marked suppression of NUMB phosphorylation and p53 upregulation, attesting to the efficacy of the aPKCζ inhibitor for prevention of p-NUMB and p53 loss (Fig. 6h ) as the most likely basis of tumor suppression. This treatment also suppressed NANOG in concordance with the positive feedback loop shown above. Treatment with the aPKCζ pseudo-substrate inhibitor in HCV NS5A Tg mice-fed AWD for 11 months resulted in >85% reduction in tumor size within 4 weeks, as assessed by micro CT examination of liver tumors. In summation, our research described the molecular mechanisms of the oncogenic activity of TBC1D15 overexpressed in tumor cells and TICs. TBC1D15 has two major tumor-promoting pathways: interference of the asymmetric division machinery by interacting with NuMA1 and disruption of NuMA1–LBN association. The latter is essential for asymmetric division, and interaction with RANGAP1, leading to AURKA–aPKCζ-induced NUMB phosphorylation and p53 degradation (Fig. 6i and Supplementary Fig. 8 ). This pathway involves TBC1D15 interaction with NOTCH/NICD resulting in NOTCH activation and stabilization. Based on this mechanistic information, we identified a small chemical inhibitor which blocked the TBC1D15–NOTCH/NICD interaction and successfully used it to prevent HCC growth in the PDX in vivo model. Lastly, the prevention of natural liver tumor formation by hepatocyte-specific TBC1D15 deficiency or NUMB mutations in NS5A Tg mice fed alcohol western diet, validated the importance of these two gene products in liver oncogenesis. 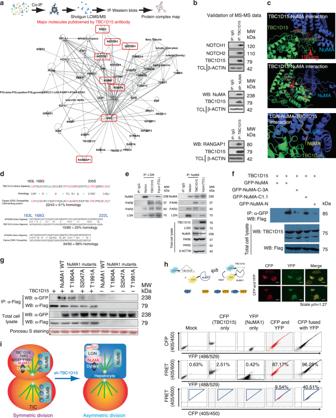Fig. 2: TBC1D15–NuMA1 interaction inhibits asymmetric cell division via inhibition of key asymmetric machinery, NuMA1–LGN interaction. aShotgun LC–MS/MS was performed on immunoaffinity purified TBC1D15-interacting proteins (highlighted in red boxes; NuMA1, RANGAP1, and NOTCH1, 2, 3, 4).bCo-immunoprecipitation-immunoblot analysis confirmed that TBC1D15 interacts with NOTCH1/2, NuMA1, and RANGAP1.cIn silico analysis predicts an interaction between TBC1D15 and NuMA1. (top) Structure model of TBC1D15 (green) binding NuMA1 (blue). (middle) Docking between TBC1D15 and NuMA1 was simulated. (bottom) TBC1D docked to NUMA with further alignment of LGN (3ro2), showing partial competition for the binding site of NUMA. TBC1D15 in green, LGN in blue, and partial NUMA in yellow.dHuman TBC1D15 protein has 51% homology withDrosophilacell fate determinant Canoe (SNO: Mammalian AFADIN homologue) that binds mammalian homologue of LGN (DrosophilaPins).eIP-Western blot analysis (left panel) and reverse IP-Western blot analysis (right panel) were performed in TBC1D15 overexpression.fDomain mapping of TBC1D15 binding domain of NuMA1 by using GFP-fused NuMA1 truncation or mutant proteins and Flag-tagged TBC1D15.gThe binding of purified flag-TBC1D15 protein with or without purified GFP-NuMA1 mutant protein was tested by in vitro binding assay.hWe performed FRET analyses between TBC1D15-CFP and NuMA1-YFP. (left upper panel) Cartoon depicting binding partners TBC1D15 and NuMA1 tagged with fluorescent proteins CFP and YFP. (left bottom panel) Living CD133+ cells transfected with the controls CFP only, YFP only, CFP and YFP as well as the CFP–YFP fusion proteins were analyzed on a FACS flow cytometer. (right panel) Representative optical images showed CFP and YFP expression in CD133+ cells with CFP and YFP. CFP is shown in red and YFP in green (Supplementary Fig.10).iHypothetical model of TBC1D15-mediated disruption of the interaction between NuMA and LGN that inhibits asymmetric cell division and promotes symmetric cell division. Source data are provided as aSource Datafile. All plasmid constructs, antibodies, recombinant proteins, recombinant DNAs, chemicals, primers, and experimental mouse models are listed in Supplementary Table 2 . Mice Liver-specific expression of NUMB-3A was achieved using tamoxifen-inducible Albumin::Cre-ERT2 for controlled targeted expression from the ROSA26 locus in hepatocytes of Ns5aTg mice. The underlying assumption for the use of Albumin::CreERT2 is that TICs are generated from albumin-expressing hepatocytes or bipotential hepatic progenitor cells. Following mice were cross-bred for 6–7 generations to produce the following genetic compound mice: Numb3A LSL [Non-phosphorylatable NUMB mutations, Numb-S7A,S265A,S284A LSL , Alb::CreERT2;Numb3A LSL , Alb::CreERT2;Numb3A LSL ;Ns5a , and Numb-3A LSL ;Ns5a ]. Successful gene knock-in was confirmed by immunoblot detection of the HA-tag of HA-NUMB-3A protein (Supplementary Fig. 7 ) in Numb3A LSL mice carrying Alb::CreERT2 which directs removal of a floxed stop signal (a tandem poly A signal) immediately downstream of the transcriptional initiation site. These mice were fed alcohol Western diet high in cholesterol and saturated fat (0.2%w/w chol, 20%Cal lard, 4%Cal corn oil, Dyets Inc.) for 12 months and injected with tamoxifen 5 times (every other day) at 2 months. A similar diet was previously shown to induce gut dysbiosis and permeability, small intestine bacterial overgrowth, and activation of TLR4 by translocated endotoxin [8] ; these sequelae promotes liver tumor formation in Ns5a Tg mice that express NS5A in liver-specific manner by ApoE -promoter [5] . FRET assays Live cells were gated according to forward and sideward scatter (FSC/SSC) and photomultiplier tube (PMT) voltages were adjusted, and FRET was evaluated in double positive cells as compensation for CFP and YFP. When excited at 405 nm, YFP showed some emission in the FRET-channel. As YFP is excited at 405 nm (FRET/YFP), an additional gate was introduced to exclude cells exhibiting false-positive signals from FRET channel. A triangular gate was introduced to FRET vs CFP was plotted and the amounts of FRET-positive cells were examined (Fig. 2h , bottom and Supplementary Fig. 10 ). The triangular gate was adjusted to measure cells transfected with CFP and YFP [34] , [35] . Immuno-affinity purification and tandem mass spectrometry We used LC-Orbitrap XL CID MS/MS to identify a potential interacting protein with TBC1D15. We did in-gel digestion of IP samples separated by SDS-PAGE. Gel pieces were then subjected to a modified in-gel trypsin digestion procedure [16] . Peptides were collected and subjected to LC–MS/MS sequencing and data analysis. The identification of TBC1D15 and its interacting proteins were carried out by mass spectrometry and validated by another functional assay. By using of strict scoring metrics, we identified several high-confidence interacting proteins, including NOTCH1, 2, 3, and 4, NuMA1, and RanGap1. RANGAP1 is a crucial regulator of RAN-GTP/GDP cycles and mitosis coordinator and known to regulate the expression of AURKA [13] . LC/MS/MS analysis For LC/MS-MS, the sample was denatured, reduced with DTT, alkylated with Iodacetamide, and digested with trypsin as described previously. Protein sequences were analyzed by use of an LC/MS system with LTQ Orbitrap XL (Thermo Fisher Scientific, San Jose, CA) and an Eksigent NanoLC Ultra 2D (Dublin, CA) as previously described [16] . Peptides were separated with 5 μm C18 beads packed in a 10 cm column (75 μm inner diameter) on a Eksigent NanoLC Ultra 2D system by use of a binary gradient of buffer A (0.1% formic acid) and buffer B (80% ACN and 0.1% formic acid). The peptides were loaded with buffer A (at a flow rate of 300 nL/min). Peptides were eluted with a linear gradient from 10 to 35% buffer B in 95 min followed by 50% B for 15 min (at a flow rate of 250 nL/min). The column was washed with 90% buffer B and equilibrated with 5% buffer B for 10 min. The eluates were sprayed into the LTQ Orbitrap XL with the ion transfer tube at 250 °C at 2.1–2.25 kV with no sheath gas flow. After accumulation to an AGC target value of 500,000 in the linear ion trap with 1 microscan, MS spectra were obtained in the orbitrap in the range of m / z 350–2000 at a FWHM resolution of 30,000. The precursors selected for fragmentation by collision-induced dissociation (CID) were processed for peptide sequencing and modification site localization. Fragment ions were examined in the linear ion trap. The five most abundant precursor ions were chosen for fragmentation by CID. The data-dependent acquisition mode was selected while five CID data-dependent MS/MS scans came after the high-resolution MS scan. For all sequencing events, dynamic exclusion was enabled to minimize repeated sequencing. Peaks selected for fragmentation more than once within 60 s were excluded from selection (10 ppm window). Data processing of LC/MS/MS Proteome Discoverer 1.4 (Thermo Fisher Scientific) was used for protein identification using Sequest algorithms. The following criteria were followed. For MS/MS spectra, variable modifications were selected to include M oxidation and C carbamidomethylation with a maximum of four modifications. Searches were conducted against Uniprot or in-house customer database. Up to two missed cleavages were allowed for the proteolytic enzyme and protease digestion. Peptides were fully tryptic. MS1 tolerance was 10 ppm. MS2 tolerance was set at 0.8 Da. If peptides met the false discovery rate of 1%, peptides reported were accepted via search engine. No fixed cutoff score threshold was in place while until the 1% FDR rate is reached, spectra were accepted. Peptides with a minimum of six amino acid lengths were processed for identification. The mass spectra were manually inspected and validated. TCGA data analyses From public datasets (TCGA, GSE17856 , GSE27150 ) of liver cancer patients showing gene expression and matched clinical data, a subset of data showing gene expression corresponding to various stages of liver cancer including metastasis was generated. The samples were divided into early stage and late metastatic stage of tumor progression to correlate the expression of Notch1 and TBC1D15 in tumor progression. A t -test was performed to estimate the differences in expression of NOTCH1 and TBC1D15 genes in early and late metastatic stage of liver cancer patients. Animal treatment These mice were fed modified high-fat Lieber–DeCarli (L–D) liquid diet (Bioserv, NJ) with alcohol (3.5%w/v) and high-fat or isocaloric dextrin using glass tubings for 3 months from 2 months of age (every day the diet is renewed). Based on the predicted incidence rates of HCC and attrition rates (15–30%) in the different genetic and dietary groups and the power analysis using the 80% power and a p -value of 0.05, the numbers of mice required for statistical analysis of the outcome in this study are derived. This formula of alcohol liquid diet has been used for many research in institutions worldwide (Lieber–DeCarli diet) and our previous study shows that the calorie intake between alcohol diet and control diet is not statistically different. aPKCζ pseudosubstrate inhibitor (PPI) One hour after a challenge (5 times a week for 4 week-treatment) on day 28, intratracheal instillation with 10 μg/mouse of aPKC ζ pseudosubstrate attached to cell permeabilization vector peptide (Tocris, Minneapolis, MO, USA) into the tumor-bearing mice (10 μg/mouse) was performed non-operatively. Inhibitor of atypical protein kinase C (aPKC) ζ is attached to cell permeabilization Antennapedia domain vector peptide. Consists of amino acids 113–129 of aPKC ζ pseudo substrate domain linked by a disulfide bridge to the Antennapedia domain vector peptide. The Antennapedia peptide is actively taken up by intact cells, at 4 or 37 °C, ensuring rapid and effective uptake of the inhibitor peptide. Once inside the cell, the disulfide bonds are subjected to reduction in the cytoplasm leading to the release of the inhibitor peptide. Induces mast cell degranulation by aPKC ζ-independent pathway. Sequence: CRQIKIWFQNRRMKWKK CSIYRRGARRWRKLYRAN* (Modifications: Disulfide bridge between 1 −1*) and RLYRKRIWRSAGR sequences (ZIP) were used as scrambled ( http://www.tocris.com/dispprod.php?ItemId=212092#.VQNbXOG2L2c ). Effect of intrathecal administration of ZIP on mechanical and thermal sensitivity or locomotor function in normal rats Intrathecal scrambled peptide (10 μg, n = 8) did not modify mechanical and thermal withdrawal responses compared to baseline in normal mice. More interestingly, intrathecal administration of 10 μg ( n = 8) of ZIP did not alter mechanical and thermal withdrawal responses compared to baseline, and the control scrambled peptide group throughout the whole experiment. Finally, neither the control scrambled peptide nor ZIP had any effect on the locomotor function of rats on the rotarod, assessed at 30 and 60 min post-injection. In vitro kinase assays Aurora A and aPKCζ were measured by SignalChem Kinase activity assay Kits as described previously. Briefly, after immuno-precipitation, samples were incubated in 20 μl reaction mixture containing each substrates and buffers. Next, 5 μl of γ-[ 32 P] ATP assay cocktail was added, the mixture was incubated in a water bath at 30 °C for 15 min. Then, 20 μl of the reaction mixture was spotted onto individual pre-cut strips of phosphocellulose p81 paper (Millipore, Temecula, CA), and the dried strips were washed 3 times with 1.0% phosphoric acid solution. Radioactivity on the p81 paper was scored in presence of scintillation fluid on a liquid scintillation analyzer (Packard Instrument Co.). The activities were presented in the figure as γ-[ 32 P] ATP specific activity or Kinase specific activity. To test if TBC1D15-mediated positive regulation of aPKCζ activity, we directly tested whether TBC1D15 increases NUMB phosphorylation in a manner dependent on aPKCζ or/and AURKA by using Huh7 cells transduced with Flag-NUMB, aPKCζ, AURKA, and/or TBC1D15 and incubated with [γ- 32 P] ATP. Following cell lysis, Flag-NUMB was immunoprecipitated and immunoblotted for autoradiography. We also treated the cells with the AURKA inhibitor MK5108 to test the contribution of this kinase. Flag-NUMB phosphorylation modestly increased with the expression of aPKCζ and AURKA but conspicuously increased with the concomitant expression of TBC1D15 and this effect was attenuated in the absence of AURKA and dose-dependently abrogated by the AURKA inhibitor MK5108. These results collectively suggest TBC1D15 positively upregulates AURKA activity and NUMB phosphorylation to drive symmetric division. NUMB phosphorylation analyses The effects on NUMB phosphorylation were assessed by incubating the cells with 32 P-orthophosphate in phosphate-free DMEM with 10% dialyzed FBS for 4 h, followed cell lysis, NUMB immunoprecipitation, PAGE, and autoradiography to monitor incorporation of 32 P into NUMB [17] . p53 dissociation from NUMB and p53 levels was assessed by co-IP and IB. Self-renewal activity was evaluated through methylcellulose spheroid formation assays and Colony formation assay as previously described [18] . In vivo mouse imaging Each month after feeding for 9 months, mice were examined for tumors by abdominal ultrasound using the VisualSonics’ Vevo 770 High-Resolution Imaging System which allows the 3D visualization and volume measurement for liver tumor mass at the Molecular Imaging Center at USC. Contrast-enhanced micro-CT and texture-based volume renderings (VRT) were performed to demonstrate a reduction of tumor size and to measure tumor volume based on 3D data collected using Inveon CT (Siemens Medical Solutions, Knoxville, TN) at a voxel size of (10 6 μm 3 ). Tumor burden was monitored monthly by measuring the body weight, which according to IACUC guidelines cannot exceed more than 5% of the control body weight. Immunoprecipitation-western blot We obtained NOTCH truncation mutants (Full-length, Δ-E, TM-RAM, RAM, and NICD) from Dr. Liang’s lab to do domain-mapping of NOTCH to interact with a trafficking protein TBC1D15 (Supplementary Table 2 ). We transfected hNOTCH1 constructs with a TBC1D15 construct to see if which domain of NOTCH1 interacts with TBC1D15. We performed IP-Western analyses to examine the interaction between TBC1D15 and NOTCH1. NOTCH1 C-20 antibody (1:1000 dilution for Western blot analyses: SIGMA) was used. In detail, Huh7 (differentiated hepatocyte-derived carcinoma cell line) were cultured in DMEM high glucose media supplemented with 10% FBS and 0.1% non-essential amino acids in T25 flask and were co-transfected with NOTCH1 full-length constructs together with TBC1D15 truncation mutants in one group and TBC1D15 full-length construct together with NOTCH1 truncation mutants in the other group. The TBC1D15 truncation mutants that were used were: Full Length mTBC1D15-FLAG, mTBC1D15 N-Terminus-FLAG, mTBC1D15-F1-2KR-FLAG, MTBC1D15-CΔC-FLAG, shTBC1D15-685 and shTBC1D15-963. NOTCH1 constructs that were used were: hNOTCH1-Full-length-myc, hNOTCH1 ΔE-3myc, hNOTCH1 TMRM-3myc, hNOTCH1ΔEΔDRAM-3myc, mNOTCH1 ΔEΔPEST-myc and hNOTCH1 ΔE V1754L. BioT was used as the transfection reagent (Bioland Scientific LLC, B01-01). Cells were lysed with Triple detergent lysis buffer after 48 h post-transfection, and half of the lysates were used for total lysate analysis while the other half were used for immunoprecipitation (IP). IP lysates were pre-cleared for 1 h with 20 μl protein A/G beads (Santa Cruz Biotechnologies, sc-2003) and incubated overnight at 4 °C with anti-flag tag (Thermo Fisher Scientific, MA1-91878) or anti-Myc tag antibody (EMD Millipore Corp, 05-274) on a rotation device. In the next day, protein A/G beads were pulled down and washed with triple detergent lysis buffer and boiled in 6× loading dye followed by electrophoresis by SDS-PAGE and protein analysis by nitrocellulose membrane. Huh7 cells were transfected with TBC1D15 full-length construct by Bio-T. The media was replaced 24 h after transfection. The cells were lysed with Triple detergent lysis buffer at 48 h post-transfection. IP lysates were incubated for 2 h in 4 °C with 1.0 µg of the appropriate control IgG (corresponding to the host species of the NuMA1 antibody, Santa Cruz Biotechnology, SC-2025) and NuMA1 antibody (BD Biosciences, 810561) on a rotation device. After 2 h, these lysates were added protein A/G beads (20 μl of 50% bead slurry) and incubated with gentle rocking for 1 h at 4 °C. Immunoprecipitates were washed with triple detergent lysis buffer and resuspended/boiled in the immunoprecipitate pellets with 10 μl 6× Laemmli sample buffer for 5 min (Supplementary Fig. 9 ). Purification of recombinant proteins To purify flag-TBC1D15, and GFP-NuMA1 wild type/mutants (T1804A, S2047A T1991A) proteins, HEK-293A cells grown to 70–80% confluence were transfected with 10 µg plasmid constructs [flag-TBC1D15, and GFP-NuMA1 wild type/mutants (T1804A, S2047A T1991A)], individually. Cells were washed once with cold PBS 48 h post-transfection, and lysed with 1 mL cold NP-40 Lysis Buffer (10 mM HEPES pH 7.5, 10 mM KCl, 1.5 mM MgCl 2 , 0.5% NP-40) for 1 h on ice, followed by centrifugation at 13,000× g for 10 min and collection of the supernatant. For each immunoprecipitation, 1 mg supernatants were incubated with 30 mL of a 40% slurry of M2 anti-Flag agarose or with 1 μg anti-GFP antibody for 2 h at 4 °C with rotating. The reaction mixture 30 µl of a 25% slurry of protein G-agarose was added, and all samples were incubated for an additional 2 h. Agarose-beads were washed once in Buffer W (20 mM Tris pH 7.3, 300 mM NaCl, 0.5% Triton X-100, 2% glycerol), washed once with PBS containing 0.2% Triton X-100, and washed once with PBS. Flag-TBC1D15 were eluted by incubation with 3× Flag peptide (1 mg/mL, Invitrogen) overnight at 4 °C with rotating. All samples were stored at −80 °C in PBS containing 5% glycerol and 1 mM DTT. In vitro protein interaction assays For purified recombinant Flag-TBC1D15, we were incubated with GFP-NuMA1 (wild type and mutants)-conjugated agarose resin for 45 min at room temperature with rotating. Samples were washed twice with Buffer W and washed once with cold PBS. Then, it was boiled in 6× Laemmle sample buffer prior to analysis by SDS-PAGE. In vitro kinase assays Kinase assays were carried out using 2 ng of the purified kinase domain of Aurora-A (Millipore Ltd., 14-511) incubated with 10 μg of the Flag-TBC1D15 and GFP-NuMA1 (wild type and mutants). The reagents were incubated for 30 min at 30 °C in kinase buffer consisting of 20 mM HEPES pH 7.5, 5 mM MgCl 2 , 0.2 M KCl, 0.5 mM EGTA, 2 mM DTT, 0.25 mM NaVO 4 , and 1 mM ATP. For the phosphorylation time-course, kinase reactions were stopped by the addition of 6× Laemmli sample buffer. To differentiate phospho-proteins from non-phosphorylated counterparts, samples were separated by Phos-TAG SDS-PAGE (Wako Pure Chemical Industries, Ltd., AAL-107). Human tissue specimens The paraffin-embedded tissue sections of human hepatocellular carcinoma (HCC) were obtained from the University of Minnesota Liver Tissue Cell Distribution System and USC cohorts. All tissue sections were obtained from patients with informed consent prior to surgery, in accordance with the approved protocol of the Institutional Review Board of the University of Minnesota, Minneapolis. The tissue sections were obtained from de-identified patients (43–67 years old) with alcohol and/or viral hepatitis associated liver tumors of varying grades. Non-tumor tissues were obtained from clearly delineated margins of surgical specimens. Immunostaining Tissue sections were re-hydrated by immersion in xylene (3 × 5 min) followed by continued re-hydration steps in 100, 90, and 70% ethanol. Following washing in PBS (3 × 5 min), antigen retrieval was performed in 10 mM sodium citrate (pH 6.0) at 90 °C for 1 h and slides were then allowed to cool down to room temperature. Following antigen retrieval, tissues were blocked in 5% goat-serum and 0.3% Triton X in BSA for overnight at 4 °C with primary antibody for TBC1D15 and NOTCH1 at 1:100 dilution ratio. Fluro-conjugated secondary antibody (Invitrogen) was added the next day at a 1:100 ratio and DAPI containing mounting media was then used to complete the staining process. Slides were then imaged using a Leica fluorescence microscope by use of the SP8 software. Dual luciferase assay Huh7 cells were treated either with sh-TBC1D15 lentivirus or with sh-Scrambled lentivirus in T25 flask. After 48 h, the cells were split into 6-well plates. Following a 24-incubation period, the cells were treated with Hey1 and Hey2 promoter constructs using BioT as the transfection reagent and transfection was done in triplicates. Constructs used were pluc Hey1, pluc Hey1 Δ215, pluc ΔSac I/Hind III, plucΔ41, PGI3-Hey2, RPBJ-mutB, and pGL-BASIC. The cells were washed in cold PBS and then lysed using passive lysis buffer after 48 h post-transfection. After lysis of the cells, the cell lysates were added to LARII reagent and then measurements were taken for firefly luciferase activity. Stop and Glo was added to stop the reaction and the Renilla Luciferase activity was measured to obtain a Firefly to Renilla ratio. Pathological analysis At the end of 12 months, the mice were euthanized and liver tumors measured, weighted, and collected for histological (H&E), biochemical (IB for TLR4, NANOG, p-NUMB, NUMB, p53, TBC1D15), and immunohistochemical (NANOG, p-NUMB, p53) analyses. 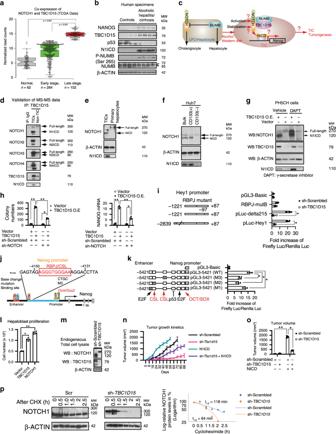Fig. 3: TBC1D15–NOTCH1 interaction promotes self-renewal and oncogenesis. aLate stage HCC patients exhibit higher NOTCH1 and TBC1D15 combined expression (TCGA): Each circle represents the expression of a single sample (p< 0.0001).bExplant liver tissues from alcoholic cirrhosis/hepatitis patients (immunoblots).cHypothetical model.dCo-IP-Western blot analyses confirmed the interaction of TBC1D15 with full-length NOTCH1/2/3/4.eImmunoblot analyses performed expression of NOCH1 and N1ICD in TICs and primary hepatocytes.fCD133+ Huh7 cells express a higher level of N1ICD compared to CD133− cells (immunoblot).gTBC1D15 overexpression elevated N1ICD in PH5CH cells (immunoblot).hColony formation (left) and expression of Nanog mRNA (right) in TBC1D15, sh-Scramble, and sh-NOTCH expressing PIL4 cells. Colony numbers were calculated as mean ± SD (n= 3). [left; *p= 0.00145 (TBC1D15 vs sh-NOTCH); **p= 0.0056 (Vector vs TBC1D15); **p= 0.01668 (sh-Scramble vs sh-NOTCH); Student’sttest].p-Values by two-tailed pairedttest. [right; *p= 0.004988 (TBC1D15 vs sh-NOTCH); **p= 0.002575 (Vector vs TBC1D15); **p= 0.02014 (sh-Scramble vs sh-NOTCH); Student’sttest].iTBC1D15 KD abrogated the activity ofHEY1promoter-luciferase in Huh7 cells. Data are represented as ±SD (n= 4).p-Values by two-tailed pairedttest. *p= 0.00953 (shTBC1D15 vs sh-Scramble; Hey1); *p= 0.018604 (sh-TBC1D15 vs sh-Scramble; Δ215); Student’sttest.jCSL-mediated Nanog activation.kSix mutant-luciferase constructs. Data are represented as ±SD (n= 3).p-Values by two-tailed pairedttest. *p= 0.008879 (WT vs M1); *p= 0.000117 (WT vs M2); *p= 0.000262 (WT vs M3) (Student’sttest).lTBC1D15 or NOTCH1 expression promotes hepatoblast proliferation. Data are represented as ±SD (n= 4).p-Values by two-tailed pairedttest. *p= 0.0001149 (Vector vs TBC1D15); **p= 0.00001853 (Vector vs NOTCH1; Student’sttest). mTBC1D15 KD reduced N1ICD but increased NOTCH1 in Huh7 cells.mCD133+ Huh7 cell lysates were analyzed for immunoblots in the presence of shRNA targeting TBC1D15 or scrambled shRNA. TBC1D15 KD reduced N1ICD but increased NOTCH1 in Huh7 cells.nTumor growth after TIC transplantation inNSGTMmice is suppressed by TBC1D15 KD. Error bars represent ±SEM.oTumor volume determined 2 months after transplantation of TICs intoNSGTMmice. Error bars represent ±SEM (n= 4).p-Values by two-tailed unpairedttest. *p= 0.00000233 (NICD vs shTBC1D15); **p= 0.0000181 (sh-Scramble vs NIICD) (Student’sttest).pTBC1D15 KD reduced NOTCH1 stability. NOTCH1 protein was immunoprecipitated and detected by immunoblotting (left). The NOTCH1 autoradiographic reading (right). Source data are provided as aSource Datafile. Non-tumor areas of the livers were also corrected for the same analyses. A pathologist with substantial experience in mouse liver histological analysis performed blind histological and immunohistochemical analysis. 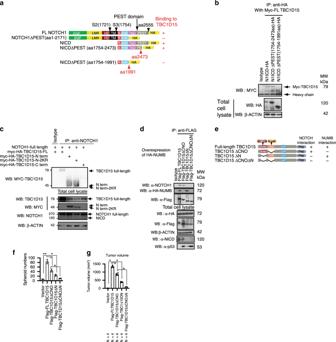Fig. 4: NOTCH1 C-terminal PEST domain interacts with N-terminus of TBC1D15 for cooperative oncogenic activity. aScheme representation of NOTCH-1 deletion mutants were generated. Co-IP-Western blot analysis identified a region between aa 2171 and aa 2473 of the PEST domain as the interaction site.bCo-IP-Western blot analysis identified interaction domains of TBC1D15 interacted with intact N1ICD-HA and N1ICDΔPEST (aa 1754–2473).cThe N-terminus but not C-terminus of TBC1D15 interacts with NOTCH-1. A similar domain mapping of TBC1D15 for its interaction with NOTCH-1 revealed aa 1–200 N-terminal fragment with known lysine residues for ubiquitination (Myc-HA-TBC1D15-N term) but not the C-terminus (Myc-HA-TBC1D15-C term), interacted with NOTCH-1. Substitution of these lysines with arginine (Myc-HA-TBC1D15-N 2KR) did not affect the binding.dCo-IP/IB showed TBC1D15–NOTCH1 interaction was lost by deletion of the N-terminus interacting domain (ΔN) while the TBC1D15–NUMB interaction was lost by deletion of the CNO domain (ΔCNO). NICD expression was lost when TBC1D15 with ΔN was expressed while p53 was restored when TBC1D15 with ΔCNO was expressed. This underscored the importance of these distinct domains for the two respective functions.eAdditional deletion analysis revealed the N-terminal domain spanning aa.163–217 upstream of the NUMB-binding Canoe (CNO) domain (aa.218–270) was responsible for TBC1D15 interaction with NOTCH.fΔCNO, ΔN, or both domains of TBC1D15 was reduced spheroid formation of PH5CH cells. Spheroid numbers were counted as mean ± SD (n= 4).p-Values by two-tailed unpairedttest. **p= 0.0001544 (Vector vs TBC1D15); *p= 0.0002660 (TBC1D15 vs ΔCNO); *p= 0.00008665 (TBC1D15 vs ΔN); *p= 0.00035214 (ΔCNO vs ΔN) (Student’sttest).gΔCNO, ΔN, or both domains incrementally contributed to the abrogation of TBC1D15-induced tumor formation (tumor pictures; left/middle and tumor volumes; right) inNSGTMmice. The visible tumors were measured at the indicated days, Error bars represent ±SD (n= 4).p-Values by two-tailed unpairedttest. **p= 0.00001448 (Vector vs TBC1D15); *p= 0.00003475 (TBC1D15 vs ΔCNO); *p= 0.00001831 (TBC1D15 vs ΔN); *p= 0.00009508 (ΔCNO vs ΔN) (Student’sttest). Source data are provided as aSource Datafile. 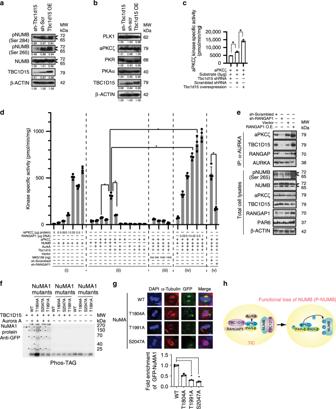Fig. 5: TBC1D15 promotes NUMB phosphorylation through RANGAP1-mediated promotion of AURKA–aPKCζ activation. aTBC1D15 knockdown inhibits NUMB phosphorylation at S265 as demonstrated by immunoblot analysis.bTBC1D15 knockdown or overexpression does not affect kinase protein levels as demonstrated by immunoblot analysis.cTBC1D15 knockdown reduces and TBC1D15 overexpression increases aPKCζ kinase activity demonstrated aby in vitro kinase assays. Data are represented as ±SD (n= 4).p-Values by two-tailed unpairedttest. *p= 0.00027596 (shTBC1D15 vs shScramble), *p= 0.000008157 (shScramble vs TBC1D15 OE) (Student’sttest).dIn vitro cell-free NUMB phosphorylation assay. Each bar represents the mean ± SD of four independent experiments.p-Values by two-tailed unpairedttest. *p= 0.000139 (TBC1D15–AURKA–aPKCζ-NUMB vs AURKA–aPKCζ-NUMB), *p= 0.0002468 (TBC1D15–AURKA–aPKCζ-NUMB vs TBC1D15-aPKCζ-NUMB), *p= 0.00000058 (TBC1D15–AURKA–aPKCζ-NUMB vs TBC1D15–AURKA–aPKCζ-NUMB-0.25μg RANGAP1), *p= 0.00008243 (TBC1D15–AURKA–aPKCζ-NUMB vs TBC1D15–AURKA–aPKCζ-NUMB-0.5 μg RANGAP1), *p= 0.0007145 (TBC1D15–AURKA–aPKCζ-NUMB-shScramble vs TBC1D15–AURKA–aPKCζ-NUMB-shRANGAP1) (Student’sttest).e(top) RANGAP1 knockdown abrogated and RANGAP1 overexpression (OE) enhances AURKA interaction with aPKCζ and TBC1D15 in Huh7 cells as determined by co-IP-Western blot analysis. (bottom) Immunoblot of total cell lysate reveals p-NUMB was reduced by RANGAP1 KD and increased by RANGAP1 OE. PAR6.fWe tested if serine or threonine residue of NuMA1 is phosphorylated by Aurora-A, and that this phosphorylation is important for association with TBC1D15. Serine or threonine residue of NuMA1 is phosphorylated by Aurora-A.gPhosphorylation of serine or threonine residue of NuMA1 by Aurora-A is important for asymmetric cell division, judged by immunofluorescence staining of α-Tubulin and NuMA1-GFP intensity. Bar graph represents fold enrichment of GFP-NuMA1. Scale bar, 10 μm. Data are represented as ±SD (n= 3).p-Values by two-tailed pairedttest. *p= 0.000667 (WT vs T1991A) *p= 0.000936 (WT vs S2047A) (Student’sttest).hHypothetical model that TBC1D15 expression promotes NUMB phosphorylation via RANGAP1–TBC1D15 interaction enhancing AURKA–aPKCζ interaction and activation. Source data are provided as aSource Datafile. 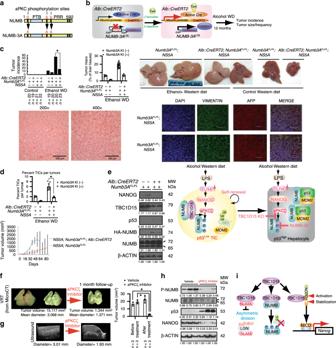Fig. 6: Targeted expression of a non-phosphorylatable mutant of NUMB reduces HCC development induced by alcohol-HCV synergism mouse model. aNon-phosphorylatable mutant of NUMB (named as NUMB-3A) was generated by serine-to-alanine substitutions of three NUMB phosphorylation sites.bThe experimental strategy of tamoxifen-inducible Cre-mediatedNUMB-3Aexpression usingAlb::CreERT2;NUMB3ALSL;NS5Amice.cIncidence of liver tumor (upper left panel), ratio of tumor mass/liver weight (%) (upper middle panel) and liver tumor pictures (upper panel, right) of the four groups of mice was decreased inAlb::CreERT2;NUMB3ALSL;NS5Amice with Ethanol WD. The visible tumors were measured at the indicated days. Error bars represent ±SEM (n= 3).pValues are shown from a chi-square test *p= 0.0003773 (chi-square test). H&E staining for mouse tumors (bottom left panel). Immunofluorescence staining of Vimentin and AFP in tumor tissues (bottom right panel). Scale bar, 30.32 μm. The representative pictures are shown from three independent experiments.d(top) The percentage of CD133+ TICs in tumor cells is compared among the four different genotypes of mice. (bottom) Tumor volume kinetics of TIC-derived tumors. The percentage of TICs of tumor cells were calculated as mean ± SD (n= 3).p-Values by two-tailed pairedttest. *p= 0.022474 (Student’sttest).e(left) Immunoblots of tumor cell lysates isolated from hepatocyte-specific expression of NUMB-3A mice. (right) Schematic presentations of LPS-activated TLR4 inducing NANOG mediated NUMB phosphorylation for p53 loss and TIC self-renewal, and of NUMB-3A-antagonism of this pathway.fMicro-CT imaging and texture-based VRT were reduced tumor size and tumor volume. The bar graph shows changes in tumor volume before and after the aPKCζ inhibitor. Error bars represent ±SEM.p-Values by two-tailed pairedttest. *p= 0.00654 (aPKCζ inhibitor; before vs after treatment), *p= 0.00095 (after treatment; vehicle vs aPKCζ inhibitor) (Student’sttest).gΤhe aPKCζ inhibitor treatment reduced liver tumors spontaneously developed in HCVNS5ATg mice fed alcohol Western diet as shown by ultrasound sonography.hImmunoblots of tumor cell lysates isolated fromNS5ATg mice fed alcohol WD of the aPKCζ inhibitor vs vehicle.iSummary of oncogenic pathways. NUMB phosphorylation and TBC1D15 are mutually required for liver tumorigenesis. Source data are provided as aSource Datafile. Reporting summary Further information on research design is available in the Nature Research Reporting Summary linked to this article.